Synthetic polymers enable non-vitreous cellular cryopreservation by reducing ice crystal growth during thawing The cryopreservation of cells, tissue and organs is fundamental to modern biotechnology, transplantation medicine and chemical biology. The current state-of-the-art method of cryopreservation is the addition of large amounts of organic solvents such as glycerol or dimethyl sulfoxide, to promote vitrification and prevent ice formation. Here we employ a synthetic, biomimetic, polymer, which is capable of slowing the growth of ice crystals in a manner similar to antifreeze (glyco)proteins to enhance the cryopreservation of sheep and human red blood cells. We find that only 0.1 wt% of the polymer is required to attain significant cell recovery post freezing, compared with over 20 wt% required for solvent-based strategies. These results demonstrate that synthetic antifreeze (glyco)protein mimics could have a crucial role in modern regenerative medicine to improve the storage and distribution of biological material for transplantation. The formation and growth of ice are highly unfavourable in most biological systems, with the exception of certain extremophiles including numerous Antarctic and Arctic fish species [1] , [2] . Ice formation and growth not only lead to mechanical damage on a cellular level, but also osmotic shock as the concentration of extracellular solutes rises as the liquid water volume fraction decreases [3] . This is a particular problem during the sub-zero storage of biological material: cryopreservation. The need to cryopreserve donated cells, tissues and organs is an escalating problem because of the burgeoning demands of regenerative medicine and organ transplantation in an aging population [4] , [5] . For example, in the United Kingdom, 6,000 units of blood are required per day, but blood can only be stored effectively for 42 days without cryopreservation and in complex isotonic solutions [6] with unacceptable rates of haemolysis in simple isotonic solutions ( Supplementary Fig. 1 ) and thus is not routinely undertaken. Cryopreservation is a time consuming and financially unviable option and necessitates the need for a continuous supply of donors, which fluctuates throughout the year [7] . In the United States of America, the waiting list for organ transplantation currently exceeds 118,000 individuals (May 2013) and with fewer than 30,000 transplants undertaken in 2012, it is imperative that no organ is wasted [8] . Nature has evolved many elegant solutions to allow life to flourish in sub-zero environments including polar oceans, where surface temperatures are regularly below −2 °C (ref. 1 ). In the circulatory system of Antarctic fish raised solute levels depress the colligative freezing point, but the observed depression cannot be explained by these solutes alone, implying a secondary component [9] , [10] . This led to the identification of antifreeze (glyco)proteins (AF(G)Ps), which are capable of further depressing the freezing point by a process known as thermal hysteresis (TH) that leaves the equilibrium melting point unchanged. Considering this, it is not surprising that soon after their discovery that these proteins were suggested as novel additives to improve the cryopreservation of cells [11] . However, there are several challenges, which have been encountered when using these materials. The first is availability as AF(G)Ps and the closely related antifreeze proteins (AFPs) can only be isolated in very small quantities from their native sources [12] . In addition, AF(G)Ps cannot be easily obtained using bacterial recombinant expression because of the required glycosylation. Furthermore, to the best of our knowledge, there are only three reported syntheses of AF(G)Ps because of the difficulty of installing the correct disaccharide moiety, and have only succeeded on a small scale [12] , [13] , [14] . The second problem is that the majority of attempts at cryopreservation using AF(G)Ps and AFPs have shown minimal benefit, and in most cases a decrease in cell recovery has been observed [11] , [15] , [16] . This has been attributed to a secondary property of AF(G)Ps known as dynamic ice shaping (DIS), which is intrinsically linked to their TH property. Essentially, AF(G)Ps bind to specific planes of ice, inhibiting their growth, but upon cooling, the remaining exposed faces grow, giving rise to a spicular (needle-like) morphology causing mechanical damage [17] . Carpenter et al. [11] and Matsumoto et al. [18] demonstrated small improvements in cryopreservation with an AFP and an AF(G)P mimic respectively, but the benefit was limited by the low concentrations, which could be applied before cell viability was reduced because of ice-shaping. Wang et al. [15] observed that AF(G)P failed to preserve rat hearts. Bovine sperm and mouse oocytes [19] appear to benefit from AFP during cryopreservation but AFPs reduce the viability of mouse sperm under similar conditions [16] . There are also indications that AF(G)Ps are cytotoxic to mammalian cells, plus the use of non-host proteins may create immunogenicity issues [20] . Upon analysis of the cryopreservation process, it has been determined that one of the major causes of cell death is actually ice recrystallization (growth) during the thawing process, rather than cell death during freezing [21] , [22] . In current cryopreservation solutions, water is replaced with an organic solvent (such as dimethyl sulphoxide (DMSO) or glycerol) and cooled rapidly to promote the formation of a glassy (ice-free) state in a process known as vitrification [21] . Devitrification upon warming (ice recrystallization) is a frequent problem, along with the intrinsic toxicity of the organic solvents that are required at very high concentrations (typically above 20 wt%) [23] , [24] . This toxicity is a problem not just for the cryopreserved cells, but also any other cells/tissue which the solvent encounters post transplantation [25] , [26] . It has therefore been hypothesized that if a compound can be identified which can achieve ice recrystallization inhibition (IRI) similar to native AF(G)Ps but without detrimental TH/DIS, then they may be able to improve vitreous cryopreservation or even allow for vitrification-free storage of cells, which would be experimentally appealing, because of the precise cooling/thawing rates required in standard protocols [3] , [27] . Ben et al. have developed a series of short glycopeptides that have specific IRI activity at very low concentrations. These analogues have been showed to be more synthetically accessible, biocompatible with human embryonic liver (WRL-68) cells and shown marginal benefits when added into standard cryopreservation solutions [28] , [29] . These peptides have also been shown to be readily internalized, making their post-thaw removal non-trivial. Current bottlenecks in the design and application of new inhibitors include a lack of mechanistic understanding into the process of IRI by AF(G)Ps and their mimetics, preventing them being translated successfully into clinical application [30] , [31] . Gibson and others have demonstrated that the non-penetrative (and hence removable post-cryopreservation) polymer poly(vinyl alcohol) (PVA) is a very potent IRI compound despite few structural similarities to AF(G)Ps, suggesting synthetic polymers can act as functional mimics of glycoproteins [32] , [33] , [34] . PVA is appealing as it is known to have minimal toxicity and is already Food and Drug Administration approved for use in dietary applications [35] . Although the reasons for activity of PVA remain unclear at present, the ongoing search for other polymeric IRIs has not identified many active candidates [31] , [36] . Other non-penetrative polymers, poly (vinylpyrrolidone) and dextran, have also been explored as cryopreservatives but have minimal IRI activity [37] , [38] . Here we show that addition of polymeric AF(G)Ps-mimics to erythrocytes enables their cryopreservation without the need for any vitrifying agents. Conventional vitrification agents such as glycerol and DMSO lead to haemolysis that must be balanced against their cryoprotective effect for clinical applications. The polymer, PVA, is shown to slow the rate of ice crystal growth during thawing, which confers protection to the erythrocytes. We report that addition of 0.1 wt% of PVA to erythrocytes enables post-freezing recovery rates of >40% for both ovine and human erythrocytes without addition of any organic solvents. Ice growth inhibition activity of synthetic polymers To demonstrate the challenges associated with addition of large volumes of conventional (organic solvent) vitrification agents used in cryopreservation [7] , [24] , [39] , both sheep and human red blood cells (RBCs) were incubated with DMSO and glycerol. Application of these solvents at 4% (v/v) and 5% (v/v), respectively, resulted in significant haemolysis ( Supplementary Fig. 2 ) even at these relatively low concentrations, below that required for successful cryopreservation. To explore the role of PVA as an AF(G)P-mimetic cryoprotectant ( Fig. 1 ), by the mechanism of inhibiting ice crystal growth during thawing, a quantitative assay was employed to demonstrate the IRI activity of PVA [40] . Briefly, a poly-nucleated ice wafer made up of ice crystals with diameters <10 μm is annealed at −6 °C for 30 min and ice crystal size reported, relative to a negative control (PBS). Figure 2 shows the IRI activity of PVA, poly (ethylene)glycol (PEG; an isomeric non-toxic polymer with no IRI activity) and the non-penetrative cryopreservative hydroxyethyl starch (HES; see also Supplementary Fig. 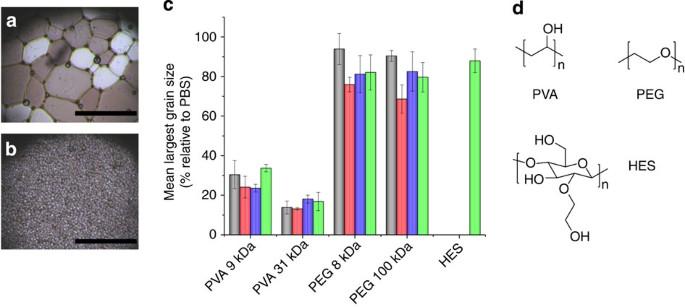Figure 2: Ice recrystallization inhibition activity of polymers. (a) Cryomicroscopic image showing native ice crystal growth in PBS following annealing at −6 °C for 30 min. (b) Cryomicroscopic image showing attenuation of ice crystal growth by the addition of 9 kDa poly(vinyl alcohol) (PVA) annealing at −6 °C for 30 min. Scale bars, 400 μm. (c) Quantitative assessment of IRI activity of polymers at 1 mg ml−1(grey), 2 mg ml−1(red), 5 mg ml−1(blue) and 10 mg ml−1(green) relative to PBS solution alone. Structures of PVA, poly (ethylene)glycol (PEG) and hydroxyethyl starch (HES) polymers are shown ind. Data presented as mean (n=3) largest grain size relative to PBS. Error bars represent±s.d. 3 for HES cryopreservation at high concentrations). PVA clearly shows potent IRI activity with arrest of ice crystal growth at concentrations as low as 0.1 mg ml −1 (~0.01 wt%), similar to native AF(G)Ps. IRI measurements over extended periods of time are shown in Supplementary Fig. 4 . In agreement with our previous reports, PEG and HES show no appreciable IRI activity at comparable concentrations, highlighting the uniqueness of PVA [34] . Additional cryomicroscopic images highlighting ice crystal growth are shown in Supplementary Fig. 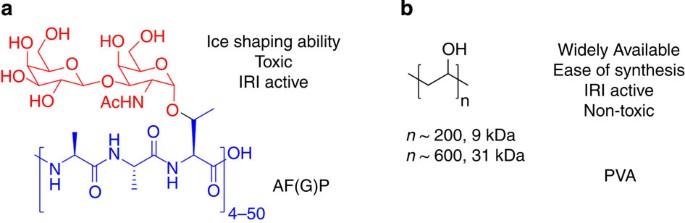5 . Figure 1: Comparison of antifreeze (glyco)protein and poly(vinyl alcohol). (a) Structure and properties of naturally occurring AF(G)Ps. (b) Structure and properties of the synthetically derived polymer PVA. IRI, ice recrystallization inhibition. Figure 1: Comparison of antifreeze (glyco)protein and poly(vinyl alcohol). ( a ) Structure and properties of naturally occurring AF(G)Ps. ( b ) Structure and properties of the synthetically derived polymer PVA. IRI, ice recrystallization inhibition. Full size image Figure 2: Ice recrystallization inhibition activity of polymers. ( a ) Cryomicroscopic image showing native ice crystal growth in PBS following annealing at −6 °C for 30 min. ( b ) Cryomicroscopic image showing attenuation of ice crystal growth by the addition of 9 kDa poly(vinyl alcohol) (PVA) annealing at −6 °C for 30 min. Scale bars, 400 μm. ( c ) Quantitative assessment of IRI activity of polymers at 1 mg ml −1 (grey), 2 mg ml −1 (red), 5 mg ml −1 (blue) and 10 mg ml −1 (green) relative to PBS solution alone. Structures of PVA, poly (ethylene)glycol (PEG) and hydroxyethyl starch (HES) polymers are shown in d . Data presented as mean ( n =3) largest grain size relative to PBS. Error bars represent±s.d. Full size image Effect of PVA and HES on ice formation Carpenter et al. [11] have demonstrated that addition of an AFP to RBCs that were cryopreserved in HES aided recovery because of inhibition of extracellular ice recrystallization, and was therefore the starting point here, but using 9 kDa PVA. HES is a non-vitrifying cryopreservative and the impact of PVA with and without HES on the ice formation/vitrification was studied by differential scanning calorimetry (DSC) and cryomicroscopy. All mixtures of HES and PVA showed a large exotherm upon cooling (rate=40 °C min −1 ) associated with homogenous ice nucleation at approximately −50 °C ( Fig. 3a,b ). Cryomicroscopy showed the formation of ice crystals in these solutions ( Fig. 3c ). As a positive control, a cryomicrograph of a 50% (v/v) solution of DMSO frozen under the same conditions is shown ( Fig. 3d ) with no ice formation (vitrified) as used in conventional cryopreservation. This proves that HES with or without PVA produces an ice-rich, rather than a vitrified state unlike organic solvent cryopreservation protocols. 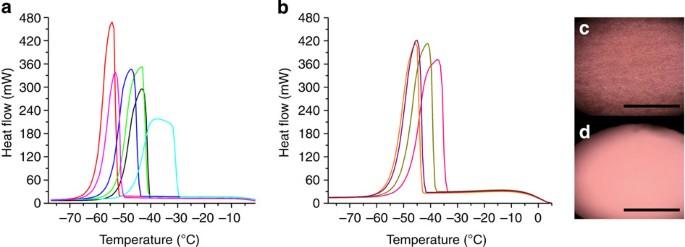Figure 3: Effect of poly(vinyl alcohol) and hydroxyethyl starch on ice formation and vitrification. (a) Differential scanning calorimetry (DSC) thermograms of 0.2 mg ml−1(black), 1 mg ml−1(red), 2 mg ml−1(green), 5 mg ml−1(dark blue), 10 mg ml−1(light blue) and 50 mg ml−1(pink) PVA in PBS. (b) DSC thermograms of mixtures of 130 mg ml−1HES+1 mg ml−19 kDa PVA (pink), 215 mg ml−1HES+1 mg ml−19 kDa PVA (orange), 130 mg ml−1HES+10 mg ml−19 kDa PVA (green) and 215 mg ml−1HES+10 mg ml−19 kDa PVA (purple), in PBS. (c) Cryomicroscopy image of a rapidly frozen sample of 10 mg ml−19 kDa PVA in PBS showing ice formation and (d) a 50% (v/v) DMSO solution with no ice present indicative of vitrification. Scale bars, 400 μm. Figure 3: Effect of poly(vinyl alcohol) and hydroxyethyl starch on ice formation and vitrification. ( a ) Differential scanning calorimetry (DSC) thermograms of 0.2 mg ml −1 (black), 1 mg ml −1 (red), 2 mg ml −1 (green), 5 mg ml −1 (dark blue), 10 mg ml −1 (light blue) and 50 mg ml −1 (pink) PVA in PBS. ( b ) DSC thermograms of mixtures of 130 mg ml −1 HES+1 mg ml −1 9 kDa PVA (pink), 215 mg ml −1 HES+1 mg ml −1 9 kDa PVA (orange), 130 mg ml −1 HES+10 mg ml −1 9 kDa PVA (green) and 215 mg ml −1 HES+10 mg ml −1 9 kDa PVA (purple), in PBS. ( c ) Cryomicroscopy image of a rapidly frozen sample of 10 mg ml −1 9 kDa PVA in PBS showing ice formation and ( d ) a 50% (v/v) DMSO solution with no ice present indicative of vitrification. Scale bars, 400 μm. Full size image Cryopreservation of sheep and human RBCs Cryopreservation of sheep RBCs in HES alone was attempted using a rapid freezing protocol to promote rapid nucleation of many (small) extracellular ice crystals, which can be tolerated by cells [21] and to prevent cellular dehydration (effect of freezing rate on ice crystal size is shown in Supplementary Fig. 6 ). Addition of large quantities of HES (215 mg ml −1 /17.7 wt%) with fast thawing temperatures (45 °C (water bath)) resulted in ~75% RBC recovery compared with 0% when conducted in PBS alone. Lowering the thawing rate by decreasing the thawing temperature to 4 or 23 °C (air) significantly reduced RBC recovery because of increased ice recrystallization (growth), which leads to osmotic and mechanical stress ( Fig. 4a ). This growth process during thawing is especially problematic for larger volumes (for example, tissues/organs) and cells, which cannot tolerate elevated thawing temperatures [23] . Despite HES being a good cryoprotectant, transfusions containing HES have been shown to elicit unacceptable side effects, including inhibition of haemostasis in vulnerable patients, which is clinically undesirable and is due to be withdrawn from clinical use [41] , [42] . Therefore, the ability of the recrystallization inhibitor, PVA, to modulate cell recovery in lower concentration HES solutions was studied. Supplementing just 10 mg ml −1 of 9 kDa PVA into 130 mg ml −1 HES resulted in a doubling of the number of recovered cells, which is a remarkable increase considering there was no noticeable effect on the freezing process, as judged by DSC or cryomicroscopy. Rather interestingly, the control experiment with just 10 mg ml −1 of 9 kDa PVA (no HES) gave rise to significant cell recovery ( Fig. 4b ). This is a remarkable observation considering the extremely low concentration applied goes against the central paradigm of using organic solvents to induce vitrification. This rather excitingly suggested that the modulation of ice growth alone might be a powerful tool to enhance cellular protection, as an alternative or supplement to classic vitrification processes. 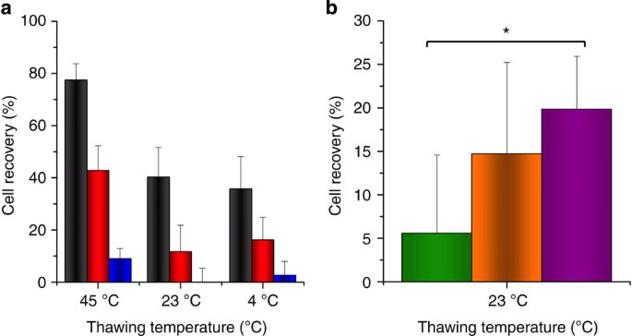Figure 4: Cryopreservation of sheep red blood cells in hydroxyethyl starch solutions. (a) Effect of thawing temperature (°C) on cell recovery. 215 mg ml−1HES (black), 130 mg ml−1HES (red) and PBS (blue). (b) Effect of supplementing (or replacing) HES with poly(vinyl alcohol) (PVA) on cell recovery. 130 mg ml−1HES (green), 130 mg ml−1+10 mg ml−19 kDa PVA (orange) and 10 mg ml−19 kDa PVA (purple). Data presented as mean (n=5) % surviving cells relative to PBS. *Statistical differenceP<0.05. Error bars represent±s.d. Figure 4: Cryopreservation of sheep red blood cells in hydroxyethyl starch solutions. ( a ) Effect of thawing temperature (°C) on cell recovery. 215 mg ml −1 HES (black), 130 mg ml −1 HES (red) and PBS (blue). ( b ) Effect of supplementing (or replacing) HES with poly(vinyl alcohol) (PVA) on cell recovery. 130 mg ml −1 HES (green), 130 mg ml −1 +10 mg ml −1 9 kDa PVA (orange) and 10 mg ml −1 9 kDa PVA (purple). Data presented as mean ( n =5) % surviving cells relative to PBS. *Statistical difference P <0.05. Error bars represent±s.d. Full size image Encouraged by the above results, PVA was explored on its own as a cryopreservative using haemolysis assays and optical microscopy. The cryopreservation of sheep RBCs with PVA, alone, showed a bell-shaped relationship between concentration and cell recovery ( Fig. 5a ). The highest recovery (40%) was found for 1 mg ml −1 of 9 kDa PVA, with recovery decreasing with both higher and lower concentrations. Biocompatibility screens show no significant haemolysis of RBCs following incubation with 9 kDa PVA at 4 °C at a concentration of 15 mg ml −1 over 6 days ( Fig. 5b ) ruling out intrinsic cytotoxicity and indicating an alternative mode of damage. 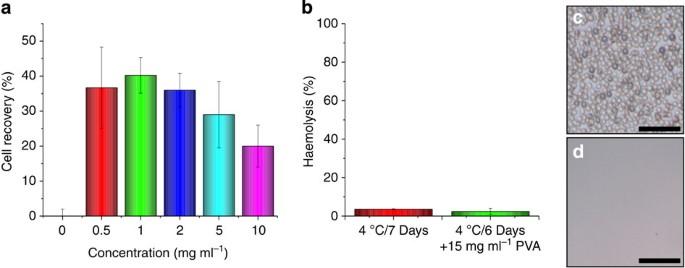Figure 5: Cryopreservation of sheep red blood cells with 9 kDa poly(vinyl alcohol). (a) RBC recovery post freeze/thaw as judged by haemolysis assay. Data presented as mean (n=5) % surviving cells relative to PBS. (b) Cytocompatibility of 9 kDa PVA. Error bars represent±s.d. Optical microscopy showing cell recovery (c) with and (d) without 10 mg ml−19 kDa PVA, post-thawing. Scale bars, 50 μm. Figure 5: Cryopreservation of sheep red blood cells with 9 kDa poly(vinyl alcohol). ( a ) RBC recovery post freeze/thaw as judged by haemolysis assay. Data presented as mean ( n =5) % surviving cells relative to PBS. ( b ) Cytocompatibility of 9 kDa PVA. Error bars represent±s.d. Optical microscopy showing cell recovery ( c ) with and ( d ) without 10 mg ml −1 9 kDa PVA, post-thawing. Scale bars, 50 μm. Full size image Previous reports have shown that high concentrations of PVA can shape ice crystals and we speculate this could explain reduced cell recovery at higher concentrations of PVA, although we did not detect this in our control experiments [43] . When higher molecular weight (31 kDa) PVA was used as a cryoprotectant significantly lower cell recovery (<10%) was observed post-thawing. Budke and Koop observed that PVA (27 kDa) at 10 mg ml −1 has notable ice-shaping activity, which agrees with this observation and our hypothesis that 31 kDa promotes DIS and that even 9 kDa PVA may have some ice-shaping effect [44] . Henceforth, the concentration and M W of PVA applied to cells is a balance between IRI and DIS. Control experiments with PEG, dextran (40 kDa) and HES (140 kDa) at similar concentrations showed essentially zero cell recovery post-freezing, demonstrating that IRI activity is essential for a polymeric cryoprotectant. In a final set of experiments, human RBCs were employed and the effect of PVA on cryopreservation was examined as a more stringent test of the technology. There are significant differences between RBCs between mammalian species in terms of membrane composition, transmembrane transporters and permeability of small molecules [45] . For example, there is a 65-fold difference between sheep and human RBCs with respect to glycerol permeability, with human RBCs having greater glycerol permeability than sheep [46] . This therefore alters their susceptibility to different forms of cryodamage because of altered rates of dehydration during freezing and thawing, which alters the probability of intracellular ice formation and vitrification. Cryopreservation experiments were conducted in an identical manner as with sheep blood, and results shown in Fig. 6 . In line with the results presented above, addition of 1 mg ml −1 of 9 kDa PVA to HES-cryopreserved RBCs resulted in a significant increase in cell recovery of around 40%, compared with what was seen for blood without PVA ( Fig. 6 ), highlighting the application to human tissue. 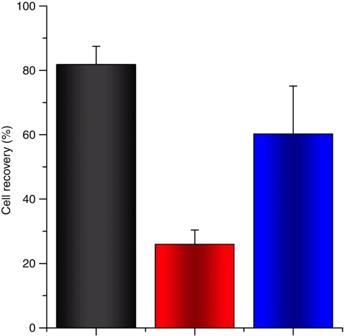Figure 6: Cryopreservation of human red blood cells in hydroxyethyl starch/poly(vinyl alcohol) solutions. Effect of thawing temperature and supplementation of 1 mg ml−19 kDa PVA in a 215 mg ml−1HES solution on cell recovery. 215 mg ml−1HES and 45 °C thaw (black), 215 mg ml−1HES and 23 °C thaw (red) and 215 mg ml−1HES+1 mg ml−19 kDa PVA and 23 °C thaw (blue). Cell recovery determined by haemolysis assays. Data presented as mean (n=5) % surviving cells relative to PBS. Error bars represent±s.d. Figure 6: Cryopreservation of human red blood cells in hydroxyethyl starch/poly(vinyl alcohol) solutions. Effect of thawing temperature and supplementation of 1 mg ml −1 9 kDa PVA in a 215 mg ml −1 HES solution on cell recovery. 215 mg ml −1 HES and 45 °C thaw (black), 215 mg ml −1 HES and 23 °C thaw (red) and 215 mg ml −1 HES+1 mg ml −1 9 kDa PVA and 23 °C thaw (blue). Cell recovery determined by haemolysis assays. Data presented as mean ( n =5) % surviving cells relative to PBS. Error bars represent±s.d. Full size image From the data presented above ( Figs 4 , 5 , 6 ), a mechanism is proposed to explain our observations ( Fig. 7 ). The first step in this protocol is rapid freezing to ensure that small extracellular ice crystals are generated (>40 °C min −1 ; Supplementary Fig. 6 ). Slow freezing rates lead to extensive ice growth and damage (mechanical and osmotic shock), unless a conventional (vitrification) approach is used [3] . These small ice crystals themselves do not cause extensive damage, until thawing when sufficient thermal energy leads to rapid recrystallization and essentially zero cell recovery ( Fig. 7bi ). Rapid thawing allows melting to occur faster than growth, overcoming this problem and hence reduced cell death ( Fig. 7bii ). Addition of PVA at relatively low concentrations (1 mg ml −1 ) limits ice crystal growth during slow thawing and results in increased cell recovery, essentially mimicking the effects of high temperature thawing without the side effects ( Fig. 7biii ). Addition of higher concentrations of PVA ( Fig. 7biv ) can also reduce ice growth, but the benefits are partially overcome by the potential secondary effects of ice shaping, which can pierce cell membranes. The key assumption here is that the PVA does not permeate the cell membrane and therefore can only influence extracellular ice. We would therefore hypothesize that, at least under the current experimental conditions, extracellular ice growth significantly contributes to cell death during freeze/thawing and is therefore an interesting target for cryopreservation modulators. The role of intracellular ice formation/growth was not probed in this study, and is likely to contribute to the <100% cell recoveries observed. 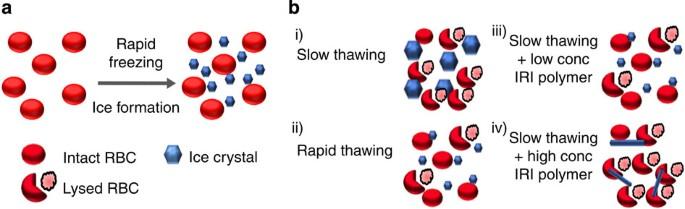Figure 7: Proposed mechanisms of cryoprotection or cell damage. (a) Initial rapid freezing step to produce large numbers of very small ice crystals. (b) Cell lysis outcomes associated with different thawing rates, the presence or absence of ice recrystallization inhibition (IRI) active additives (poly(vinyl alcohol)) and the effect of IRI concentration. RBC, red blood cell. Figure 7: Proposed mechanisms of cryoprotection or cell damage. ( a ) Initial rapid freezing step to produce large numbers of very small ice crystals. ( b ) Cell lysis outcomes associated with different thawing rates, the presence or absence of ice recrystallization inhibition (IRI) active additives (poly(vinyl alcohol)) and the effect of IRI concentration. RBC, red blood cell. Full size image In this communication, we demonstrate that polymeric mimics of AF(G)Ps are extremely potent modulators of ice crystal growth during the thawing of frozen cellular samples. The polymer used here, PVA, has excellent biocompatibility and was shown to confer protection to RBCs at concentrations as low as 1 mg ml −1 or 0.1 wt%. This is remarkably low (400 × less than glycerol) and demonstrates that it is possible to reproduce the most desirable properties of AF(G)Ps, without reproducing its exact structure, which is especially important considering the low supply, difficult synthesis and high price of AF(G)Ps. We demonstrate that during the freezing process, there is significant ice formation in the cryopreservation solution, which challenges the central dogma of this field, which is to prevent ice formation through addition of toxic glass-forming solvents such as glycerol. Complimentary physicochemical analysis by cryomicroscopy and DSC supports these observations. Considering the urgent medical need for an improved technique to bank, distribute and transplant human cells and tissues this approach could have a significant impact on human health. Future work will focus on optimization of this system, as well as investigations with a wide range of cells and tissues. Preparation of cryopreservatives 9 kDa PVA (average M w =9,000–10,000, 80% hydrolysed), 31 kDa PVA (average M w =31,000–50,000, 98–99% hydrolysed), 8 kDa PEG (average M w =8,000) and 100 kDa PEG (average M w =100,000) were sourced from Sigma-Aldrich, UK. HES was isolated from Volulyte (Fresenius Kabi Ltd, Runcorn, UK). Before use, all polymers were purified by dialysis (4 l H 2 O with at least 5 changes) against 1,000 MWCO membranes (Spectrum Laboratories Inc., CA, USA) to remove any small molecule contaminants. Samples were then freeze dried under vacuum overnight and then diluted in PBS to the final concentrations required. IRI activity To demonstrate IRI activity, a modified ‘splat’ assay was conducted [40] . A 10-μl droplet is dropped 1.8 m onto a coverslip (no. 0 thickness) pre-cooled on a CO 2(s) chilled aluminum plate forming a polynucleated wafer of ice crystals (each ice crystal is <10 μm). The coverslip is immediately transferred to a Linkam BCS196 (N 2(l) cooled) cryostage (Linkam Scientific Instruments Ltd, Guildford, UK) and annealed at −6 °C for 30 min (or longer when specified). Afterwards, the wafers are imaged using an Olympus CX41 microscope equipped with a UIS-2 10x/0.25/∞/-/FN22 lens (Olympus Ltd, Southend on sea, UK) and a Canon EOS 500D SLR digital camera (Canon (UK) Ltd, Surrey, UK) through crossed polarisers. The sizes of the ten largest crystals were measured using the freely available image-processing software ImageJ ( http://rsbweb.nih.gov/ij/index.html ) and the mean largest grain size expressed as a percentage of a PBS control. DSC DSC assessment of ice formation and vitrification was performed with a range of HES and PVA mixtures. 40 μl aluminium pans and samples (15 μl) were accurately weighed to ±0.01 mg and transferred to a DSC-1 STAR e System (Mettler-Toledo Ltd, Leicester, UK). Heat flow (mW) was measured and recorded against an empty pre-weighed 40 μl aluminium reference pan starting from 5 to −78 °C at 40 °C min −1 with the presence of a large exotherm demonstrating ice formation. Cryomicroscopy Cryomicroscopy was undertaken using a Linkam BCS196 (N 2(l) cooled) cryostage (Linkam Scientific Instruments Ltd) coupled to an Olympus CX41 microscope equipped with a UIS-2 10x/0.25/∞/-/FN22 lens (Olympus Ltd) and a Canon EOS 500D SLR digital camera (Canon (UK) Ltd). A 5 μl sample was placed between two coverslips (No. 0 thickness) and cooled rapidly from 5 to −78 °C at 40 °C min −1 for a range of solutions and viewed in real time for ice formation/vitrification. Samples that were negative for ice formation at −78 °C were repeated with the final temperature lowered further to −150 °C each of which were still negative for ice formation. RBC preparation Sheep RBCs (defibrinated, packed cell volume between 32–52%) were purchased on demand from TCS Biosciences Ltd, Buckinghamshire, UK. Human RBCs were donated by healthy volunteers and collected in EDTA vacutainers. Both samples were prepared identically with cells centrifuged (1,950 g , 5 min, 25 °C) and the top layer (containing any residual plasma and its constituents) removed and replaced with an equal volume of PBS. When not in use cells were stored in this form at 4 °C for a maximum of 7 days. Experiments with human RBCs had local ethical approval (Coventry Research Ethics Committees 07/ H1210/141) with all patients involved having given written informed consent. Measurement of RBC haemolysis and cell recovery A 40 μl aliquot of the desired RBC suspension was added to 400 μl PBS and centrifuged (1,000 g , 5 min, 4 °C) to remove intact cells. 50 μl of the supernatant was added to 150 μl of PBS in a 96-well plate and an absorbance measurement at 450 nm recorded to assess the extent of haemolysis and cell recovery. Hundred percent haemolysis samples were prepared by osmotic shock through addition of 500 μl H 2 O to a 500 μl RBC suspension that was vortexed vigorously and cryopreserved with an absence of cryoprotectant and thawed slowly, inciting total haemolysis. Control (0% haemolysis) samples were prepared by the addition of 500 μl PBS to a 500 μl RBC suspension and left untreated at 23 °C for 60 min. Cell recovery was calculated by subtracting the attained haemolysis (%) from 100 (%) giving a figure for cell recovery (%). RBCs cryopreservation at varied thawing rates A 50 μl aliquot of prepared RBCs (packed cell volume between 32 and 52%) with samples were prepared in quintuplet was added to 50 μl of cryoprotectant (HES/9 kDa PVA) in PBS in 1.8 ml cryovials and vortexed gently giving a final pack cell volume between 16 and 26%. Each sample was then rapidly frozen in an isopropanol/CO 2(s) bath (−78 °C) for 60 s and subsequently stored in CO 2(s) for 20 min. Samples were allowed to thaw at the desired temperature (4 °C (air), 150 min; 23 °C (air), 30 min; 45 °C (water bath), 10 min) before cell recovery was measured as previously described. Cryopreservation of RBCs with PVA A 500 μl aliquot of prepared RBCs (samples were prepared in quintuplet) was added to 500 μl of 9 kDa PVA in PBS in 1.8-ml cryovials and mixed by inversion. Each sample was then rapidly frozen in an isopropanol/CO 2(s) bath (−78 °C) for 60 s and subsequently stored in CO 2(s) for 20 min. Samples were allowed to thaw at 23 °C (air) for 30 min before cell recovery was measured as previously described. Cytotoxicity of glycerol and DMSO The cytotoxicity of DMSO and glycerol to ovine and human RBCs was tested as follows: 500 μl aliquots of RBCs (samples were prepared in quintuplet) were added to 500 μl 2 × final concentration DMSO/glycerol in PBS and mixed by inversion. The samples were incubated (200 r.p.m., 23 °C) for the desired period of time before immediate assessment of haemolysis. Concentrations of DMSO from as low as 0.5% (v/v) after 150 min and 1.5% (v/v) after 60 min began to show significant haemolysis. Glycerol at a concentration of 5% (v/v) showed near total haemolysis after 15 min with ovine erythrocytes. Data analysis All statistics and calculations for (%) haemolysis, (%) cell recovery and (%) mean largest grain size were determined using Microsoft Excel 2008 for Mac. Significance determination for cryopreservation data used a two-tailed homoscedastic Student’s t -test with a 95% confidence interval. Assessment of ice crystal formation Freezing is highly dependant upon the rate of cooling. This can be easily exemplified using cryomicroscopy by cooling non-vitrifying samples at a variety of rates. A 5-μl droplet of PBS was placed between two (no.0 thickness) 19-mm diameter coverslips and was cooled to +2 °C. The sample was then cooled to −80 °C at one of a variety of cooling rates and images taken at × 200 magnification at a focal plane showing ice formation. The same sample was used in each instance and heated rapidly to +10 °C for 2 min to ensure all ice was melted between cooling cycles. How to cite this article: Deller, R. C. et al. Synthetic polymers enable non-vitreous cellular cryopreservation by reducing ice crystal growth during thawing. Nat. Commun. 5:3244 doi: 10.1038/ncomms4244 (2014).